Vascular channels formed by subpopulations of PECAM1+melanoma cells Targeting the vasculature remains a promising approach for treating solid tumours; however, the mechanisms of tumour neovascularization are diverse and complex. Here we uncover a new subpopulation of melanoma cells that express the vascular cell adhesion molecule PECAM1, but not VEGFR-2, and participate in a PECAM1-dependent form of vasculogenic mimicry (VM). Clonally derived PECAM1 + tumour cells coalesce to form PECAM1-dependent networks in vitro and they generate well-perfused, vascular endothelial growth factor (VEGF)-independent channels in mice. The neural crest specifier AP-2α is diminished in PECAM1 + melanoma cells and is a transcriptional repressor of PECAM1. Re-introduction of AP-2α into PECAM1 + tumour cells represses PECAM1 and abolishes tube-forming ability, whereas AP-2α knockdown in PECAM1 − tumour cells upregulates PECAM1 expression and promotes tube formation. Thus, VM-competent subpopulations, rather than all cells within a tumour, may instigate VM, supplant host-derived endothelium, and form PECAM1-dependent conduits that are not diminished by neutralizing VEGF. Solid tumours require blood vessels for growth, access to oxygen and nutrients, and the removal of waste products. Thus, Folkman proposed that anti-angiogenic therapies could be used to attack tumour-associated blood vessels and shrink solid tumours [1] . Anti-angiogenic therapies are typically designed to target vascular endothelial cells (ECs) that form tumour blood vessels. Therefore, anti-angiogenic drugs should be active against a spectrum of cancers. Furthermore, unlike conventional cytotoxic chemotherapy that targets genetically unstable and heterogeneous tumour cells, anti-angiogenic therapies target the vasculature that theoretically will not acquire drug resistance but should respond predictably to angiogenesis inhibition. Whereas numerous preclinical models have documented the successful use of angiogenesis inhibitors to block tumour growth, these studies collectively show that tumours are typically only growth delayed, rather than driven into dormancy [2] , [3] , [4] , [5] . Thus, the tumour vasculature may be more complex than previously considered and tumours may have secondary mechanisms for re-vascularization [6] , [7] . For example, freshly isolated tumour-specific EC (TEC) from different tumour types display multiple abnormalities [8] , [9] , [10] , [11] , [12] . Two tumour-specific modes of neovascularization including ‘transdifferentiation’ of stem-like tumour cells and vasculogenic mimicry (VM) are also suggested [13] , [14] , [15] , [16] , [17] , [18] , [19] , [20] , [21] , [22] . These tumour cell autonomous routes to neovascularization may underlie some of the dysfunctional features of tumour blood vessels and create outlets for escape from angiogenesis inhibition. VM, initially described in aggressive forms of uveal melanoma, has been documented in multiple tumour types and is correlated with poor patient survival [23] . Tumour cell-lined networks are typically identified in histological sections by periodic acid-Schiff staining of matrix-rich channels, which contain blood, with few or no EC present. However, the different molecular mechanisms that generate VM-competent tumour cells are unclear and how tumour cell-lined conduits are formed and connected with the host vasculature is undetermined. Furthermore, it remains controversial whether tumour cells actively engage tumour blood vessels in a process resembling EC-mediated angiogenesis or if tumour cells simply fill in gaps between neighbouring EC in a passive, nonfunctional manner [24] . Bona fide TEC may be identified and isolated from collagenase-dispersed tumours using intercellular adhesion molecule-2 (ICAM2) or platelet EC adhesion molecule (PECAM1, also known as CD31) antibodies followed by immunomagnetic separation [8] , [25] . Using this methodology, we have uncovered a novel subpopulation of PECAM1 + tumour cells in melanoma that participate in a PECAM1-dependent form of VM. Unlike previous models suggesting that tumour cells contribute to neovascularization through endothelial-like differentiation or recapitulation of developmental plasticity, we demonstrate that VM-competent tumour cells exist as stable, yet hidden subpopulations in heterogeneous melanomas [15] , [26] , [27] . Clean separation of PECAM1 − and PECAM1 + clonal populations from the same tumour has allowed us to compare and contrast the differential roles these two populations have during tumour growth, angiogenesis and responses to anti-angiogenic therapy. Identification of PECAM1 + tumour cells from B16F10 melanoma Using PECAM1 immunomagnetic separation of collagenase-dispersed B16F10 melanoma allografts [8] , [28] , we enriched a PECAM1 + population to ~98% purity, as determined by flow cytometry ( Fig. 1a,b ). Compared with the PECAM1 − fraction, the enriched PECAM1 + population expressed abundant Pecam1 mRNA by semi-quantitative reverse transcription (RT)–PCR ( Fig. 1c ). Unexpectedly, VE-cadherin mRNA was not detected in the PECAM1 + fraction, in contrast to mouse dermal ECs (mECs) used as a positive control ( Fig. 1c ) [8] . However, the PECAM1 + fraction strongly expressed the melanocyte marker tyrosinase (Tyr) leading us to suspect that we had enriched a previously unidentified PECAM1 + subpopulation of melanoma cells from the B16F10 cell line. To test this possibility, we engrafted parental B16F10-GFP tumour cells into wild type, C57BL/6 mice and unlabelled B16F10 cells into C57BL/6-Tg (CAG-EGFP) 1Osb/J mice. We then used PECAM1 immunomagnetic separation to retrieve highly purified fractions as before. The results showed that B16F10-GFP tumour cells in a wild-type host generated PECAM1 + /GFP + cells, whereas wild-type tumours in a green fluorescent protein (GFP) host generated PECAM1 + /GFP − cells ( Fig. 1d ). These results are consistent with a tumour cell-of-origin for the PECAM1 + cells we have isolated. Furthermore, these results appear to rule out the possibility of fusion between tumour cells and PECAM1 + vascular EC in this particular mouse tumour model. 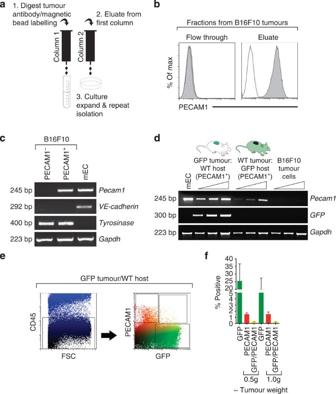Figure 1: Identification, isolation and characterization of PECAM1+tumour cells from B16F10 melanoma. (a) PECAM1 antibodies coupled to immunomagnetic beads were used to enrich PECAM1+tumour cells from collagenase-digested B16F10 tumours. (b) The enriched cells (eluate) are ~99% PECAM1+by flow cytometry. (c) Purity of the cells was further confirmed by semi-quantitative RT–PCR. The PECAM1+fraction from B16F10 expresses Pecam1 and Tyr, but not VE-cadherin. (d) Retrieval of PECAM1+/GFP+cells from GFP tumours engrafted in wild-type (WT) hosts and PECAM1+/GFP−cells engrafted in GFP hosts. Following immunomagnetic separation with PECAM1 antibodies, increasing amounts of cDNA template were analysed by semi-quantitative RT–PCR, indicated by the wedge. (e) Detection of PECAM1+/GFP+tumour cellsin vivoafter injecting B16F10-GFP tumour cells into WT hosts. CD45+haematopoietic cells were excluded by out-gating. The upper right quadrant are PECAM1+tumour cells, which comprise ~0.1% of each tumour. (f) The percentage of PECAM1+/GFP+tumour cells are shown for two time points when tumours were different sizes (n=3 mice per group; error bars=s.e.m.). Figure 1: Identification, isolation and characterization of PECAM1 + tumour cells from B16F10 melanoma. ( a ) PECAM1 antibodies coupled to immunomagnetic beads were used to enrich PECAM1 + tumour cells from collagenase-digested B16F10 tumours. ( b ) The enriched cells (eluate) are ~99% PECAM1 + by flow cytometry. ( c ) Purity of the cells was further confirmed by semi-quantitative RT–PCR. The PECAM1 + fraction from B16F10 expresses Pecam1 and Tyr, but not VE-cadherin. ( d ) Retrieval of PECAM1 + /GFP + cells from GFP tumours engrafted in wild-type (WT) hosts and PECAM1 + /GFP − cells engrafted in GFP hosts. Following immunomagnetic separation with PECAM1 antibodies, increasing amounts of cDNA template were analysed by semi-quantitative RT–PCR, indicated by the wedge. ( e ) Detection of PECAM1 + /GFP + tumour cells in vivo after injecting B16F10-GFP tumour cells into WT hosts. CD45 + haematopoietic cells were excluded by out-gating. The upper right quadrant are PECAM1 + tumour cells, which comprise ~0.1% of each tumour. ( f ) The percentage of PECAM1 + /GFP + tumour cells are shown for two time points when tumours were different sizes ( n =3 mice per group; error bars=s.e.m.). Full size image Next, we determined the proportion of PECAM1 + tumour cells in B16F10 tumours in vivo using flow cytometry. Tumours were harvested once they had reached ~0.4 g (±0.26 g, s.e.m.) or~1.0 g (±0.22 g, s.e.m.) in size. The proportion of PECAM1 + tumour cells remained at ~0.2% of the total cellular pool, irrespective of tumour size. After gating out CD45 + haematopoietic cells, the ratio of PECAM1 + vascular EC to PECAM1 + tumour cells was approximately 10:1 ( Fig. 1e,f ). Taken together, these results suggest that subpopulations of melanoma cells may express the vascular cell adhesion molecule PECAM1 in vivo . Isolation of PECAM1 + clones from B16F10 melanoma PECAM1 + cells comprised a minor fraction of B16F10 cultures and could not be easily detected by flow cytometry. However, occasional clusters of PECAM1 + cells could be found under fluorescence microscopy when B16F10 cultures were directly stained with PECAM1 antibodies ( Supplementary Fig. 1a ). To further explore the significance and biological functions of PECAM1 + melanoma cells, we prepared clonal populations using limiting dilution assays from highly enriched PECAM1 + fractions ( Fig. 2a ). In 50% enriched fractions, PECAM1 + tumour cells were visible as large, flattened colonies that were distinct in appearance from spindle-shaped, PECAM1 − tumour cells ( Supplementary Fig. 1b ). These PECAM1 + tumour cells could be cleanly separated from their PECAM1 − counterparts using cloning rings or multiple rounds of immunomagnetic separation with PECAM1 antibodies followed by limiting dilution assays. Quantitative PCR (qPCR) using clonally derived populations revealed robust Pecam1 mRNA expression in clones A2 and A5 but not in clone A1 ( Fig. 2b ). No mRNAs were detected for VE-cadherin or Vegfr-2 in PECAM1 − or PECAM1 + tumour cells. Tyr was expressed by all melanoma cells but not mEC, as expected. Confocal microscopy revealed that PECAM1 was concentrated at the cell membrane in mEC but was diffusely localized at the membrane and throughout the cytoplasm in PECAM1 + tumour cells ( Supplementary Fig. 1c ). Western blotting confirmed a migrating band at the expected size for murine PECAM1 in PECAM1 + clones ( Fig. 2c ). PECAM1 was tyrosine phosphorylated in PECAM1 + tumour cells suggesting it may have similar signalling abilities in both EC and tumour cells ( Supplementary Fig. 1d ). 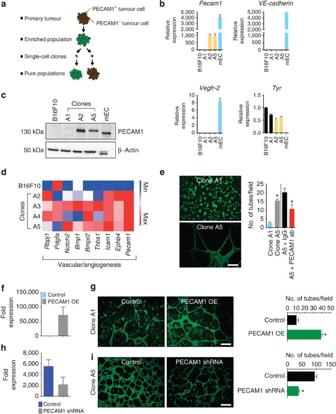Figure 2: PECAM1+clonally derived populations from B16F10 melanoma display vascular characteristics and form PECAM1-dependent tube-like structures. (a) Strategy for preparation of PECAM1+clonal populations from B16F10 melanoma using limiting dilutions of partially enriched cellular fractions. (b) Characterization of PECAM1−and PECAM1+clonal populations using qPCR. (c) Western blotting for PECAM1 using whole-cell extracts from the indicated cell type. PECAM1 migrates at the expected size of ~130 kDa. Blots were stripped and re-probed with β-actin antibodies to show equal loading. (d) Microarray analysis of parental B16F10 and PECAM1+clonal populations derived from B16F10. Only known vascular or angiogenesis-related genes shown to be upregulated in PECAM1+clones are shown. (e) Images from tube-forming assay in Matrigel comparing a PECAM1−(A1) and PECAM1+(A5) clone. Tube-like structures in high-power fields were quantified and plotted. Sample means were statistically significant as determined by a Student’st-test (P<0.02,n=6 wells per condition). (f) qPCR analysis ofPecam1expression in PECAM1−melanoma cells (clone A1) following ectopic PECAM1 expression. (g) Images of control-transfected cells and PECAM1 overexpressing (OE) cells are shown after a 16-h tube formation assay and quantified at right. Means are statistically significant as determined by a Student’st-test (P<0.001,n=6–7 wells per condition). (h) qPCR analysis ofPecam1expression in PECAM1+melanoma cells (clone A5) following short hairpin RNA (shRNA) knockdown. (i) Images of empty-vector transfected andPecam1shRNA-transfected cells are shown after a 16-h tube formation assay and quantified at right. Means are statistically significant as determined by a Student’st-test (P<0.001,n=7–8 wells per condition; scale bars, 100 μm, error bars=s.e.m.). Figure 2: PECAM1 + clonally derived populations from B16F10 melanoma display vascular characteristics and form PECAM1-dependent tube-like structures. ( a ) Strategy for preparation of PECAM1 + clonal populations from B16F10 melanoma using limiting dilutions of partially enriched cellular fractions. ( b ) Characterization of PECAM1 − and PECAM1 + clonal populations using qPCR. ( c ) Western blotting for PECAM1 using whole-cell extracts from the indicated cell type. PECAM1 migrates at the expected size of ~130 kDa. Blots were stripped and re-probed with β-actin antibodies to show equal loading. ( d ) Microarray analysis of parental B16F10 and PECAM1 + clonal populations derived from B16F10. Only known vascular or angiogenesis-related genes shown to be upregulated in PECAM1 + clones are shown. ( e ) Images from tube-forming assay in Matrigel comparing a PECAM1 − (A1) and PECAM1 + (A5) clone. Tube-like structures in high-power fields were quantified and plotted. Sample means were statistically significant as determined by a Student’s t -test ( P <0.02, n =6 wells per condition). ( f ) qPCR analysis of Pecam1 expression in PECAM1 − melanoma cells (clone A1) following ectopic PECAM1 expression. ( g ) Images of control-transfected cells and PECAM1 overexpressing (OE) cells are shown after a 16-h tube formation assay and quantified at right. Means are statistically significant as determined by a Student’s t -test ( P <0.001, n =6–7 wells per condition). ( h ) qPCR analysis of Pecam1 expression in PECAM1 + melanoma cells (clone A5) following short hairpin RNA (shRNA) knockdown. ( i ) Images of empty-vector transfected and Pecam1 shRNA-transfected cells are shown after a 16-h tube formation assay and quantified at right. Means are statistically significant as determined by a Student’s t -test ( P <0.001, n =7–8 wells per condition; scale bars, 100 μm, error bars=s.e.m.). Full size image PECAM1 + melanoma cells generate PECAM1 + progeny We found that PECAM1 expression in PECAM1 + clones was stable in vitro and was not diminished by growth in different culture media ( Supplementary Fig. 2a ). However, cell-surface PECAM1 was reduced by >50% when PECAM1 + tumour cells were detached from tissue culture dishes using trypsin as opposed to accutase, which does not affect PECAM1 surface expression ( Supplementary Fig. 2b ). In addition, routine passaging of cells did not diminish PECAM1 expression ( Supplementary Fig. 2c ). Interestingly, PECAM1 + tumour cells displayed a slight growth delay in vitro and in vivo when engrafted into mice ( Supplementary Fig. 2d ). Long-term in vitro propagation of PECAM1 − and PECAM1 + tumour cells revealed that PECAM1 + tumour cells generally give rise to PECAM1 + progeny and vice versa ( Supplementary Fig. 2e ). To determine the fate of PECAM1 − and PECAM1 + tumour cells in vivo , we transduced PECAM1 + and PECAM1 − tumour cells with GFP using lentivirus to generate PECAM1 + /GFP + (clone A5) or PECAM1 − /GFP + (clone A1) lines. We then injected 1.0 × 10 6 tumour cells subcutaneously in wild-type C57BL/6 mice. Flow cytometry of collagenase-dispersed tumours revealed that, in general, PECAM1 + tumour cells generate PECAM1 + progeny, whereas PECAM1 − tumour cells generate mostly PECAM1 − progeny ( Supplementary Fig. 2f ). When quantified by flow cytometry, PECAM1 − tumours generated a mixed population consisting of ~2% PECAM1 + progeny and ~98% PECAM1 − progeny. These results suggest that PECAM1 − and PECAM1 + melanoma cells are stable subpopulations but may generate their counterparts at low frequencies with a tendency for PECAM1 − tumour cells to generate PECAM1 + progeny. Finally, karyotypes performed on PECAM1 + and PECAM1 − clones showed that PECAM1 − tumour cells were more variable in chromosome counts with a median chromosome number of 70, whereas PECAM1 + tumour cells had a median chromosome count of 64 ( Supplementary Fig. 3a,b ). Both PECAM1 − and PECAM1 + clones displayed similar marker chromosomes to those observed in previously published reports of the B16 cell line [29] , [30] . This result, in addition to the shared chromosomal aberrations between the two populations, suggests that the PECAM1 + fraction may have persisted and been continuously generated at a low frequency within the B16F10 cell line for decades. In vitro vascular properties of PECAM + melanoma To further characterize established PECAM1 + clones, we carried out a microarray analysis using an Affymetrix mouse gene ST1.0 platform. A complete microarray data set showing differentially expressed genes in PECAM1 − and PECAM1 + tumour cells has been uploaded to the Gene Expression Omnibus. Notably, microarray analysis showed an enrichment of additional candidate genes associated with known vascular functions in PECAM1 + clones (A2, A3, A4, A5) compared with parental B16F10 tumour cells. These genes included Ephb4, Bmpr2, Pdgfa, Icam1 (CD54), Thbs1, Bmp1, Rbpj1 and Notch2 ( Fig. 2d ). Expression of these genes was confirmed by qPCR ( Supplementary Fig. 4 and see Supplementary Table 1 for a complete list of PCR primer sets). Because PECAM1 is a cell adhesion molecule known to mediate in vitro tube formation of bona fide EC, we assessed whether PECAM1 + melanoma cells might also undergo in vitro tube formation [31] , [32] . PECAM1 + tumour cells displayed a four- to fivefold increase in branching tube-like networks compared with their PECAM1 − counterparts. PECAM1 − tumour cells only formed occasional tube-like structures, which were not stable in culture. Tube-like structures in PECAM1 + tumour cells could be inhibited by ~50% using a PECAM1-blocking antibody indicating a functional role for PECAM1 in this assay ( Fig. 2e ) [33] . Gain of function experiments showed that PECAM1 overexpression in PECAM1 − tumour cells (clone A1) stimulated in vitro tube formation approximately fourfold, whereas PECAM1 short hairpin RNA in PECAM1 + tumours cells (clone A5) diminished tube formation by ~50% ( Fig. 2f–i ). These results suggest that PECAM1 is a marker of a unique subpopulation of B16F10 tumour cells and it plays a functional role in the establishment and stability of in vitro tube-like networks. PECAM1 + tumour cells exist in spontaneous murine melanoma Next, we turned to the ΔBraf/Pten −/− genetically engineered mouse model of melanoma to assess whether PECAM1 + tumour cells were present in spontaneous tumours ( Fig. 3a ) [34] . First, we measured Pecam1 mRNA expression using qPCR in two cell lines recently derived from tumours in ΔBraf/Pten −/− mice [35] . The results showed that Pecam1 mRNA levels were above the zero transcript threshold we established using a known PECAM1 − clone derived from B16F10 (clone A1; Fig. 3b ). These results suggested that, similar to B16F10, a minor subpopulation of PECAM1 + tumour cells might be present within ΔBraf/Pten −/− tumour cells. To address this possibility, we used PECAM1-mediated immunomagnetic enrichment in PBT2460 tumour cells and found that after six enrichment steps, about 15% of the population expressed PECAM1 on the cell surface by flow cytometry. After two additional enrichment steps, about 98% of the population expressed PECAM1 ( Fig. 3c ). qPCR confirmed an ~100-fold increase in Pecam1 mRNA in the enriched fraction when compared with the un-enriched parental population but VE-cadherin and Vegfr-2 were absent from both populations ( Fig. 3d ). Notably, these PECAM1 + cells derived from ΔBraf/Pten −/− tumours were not identical to those obtained from B16F10; namely, unlike PECAM1 + cells from B16F10 melanoma, they did not express ICAM1 protein or mRNA by qPCR ( Supplementary Fig. 5a,b ). 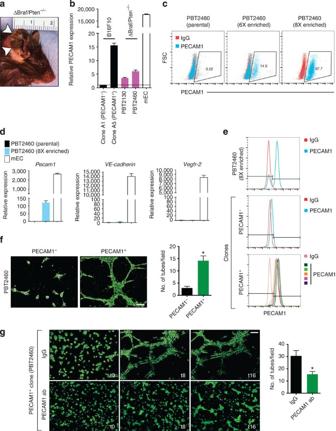Figure 3: PECAM1+/VEGFR-2−tumour cells exist in a genetically engineered mouse model of melanoma and they form vascular-like networks in Matrigel. (a) Examples of tumours from ΔBraf/Pten−/−mice. (b) qPCR analysis ofPecam1expression in PECAM1−and PECAM1+B16F10 clonal populations and two additional unsorted cell lines derived from dispersed tumours from ΔBraf/Pten−/−mice. mEC are a positive control forPecam1expression. (c) Flow cytometry analysis of unsorted (parental) PBT2460 cells shows ~3% positivity for PECAM1. After six rounds of PECAM1 selection, this fraction increases to ~15% and after eight rounds to ~98%. (d) qPCR analysis of the parental PBT2460 population versus the 8X-enriched fraction. BasalPecam1expression is ~100-fold higher in the 8X-enriched fraction compared with unsorted PBT2460 cells, whereas neither population expressesVE-cadherinnorVegfr-2. (e) Using the 8X-enriched fraction, single-cell clones were prepared by limiting dilution assays and then analysed by flow cytometry for PECAM1 expression. (f) Clonally derived PECAM1+PBT2460 cells show an ~5-fold increase in tube formation as compared with PECAM1−cells. Sample means were statistically significant as determined by a Student’st-test (P<0.0001). (g) Time-lapse images of tube formation assay using clonally derived PECAM1+PBT2460 cells incubated with either a nonspecific IgG (top row) or PECAM1-blocking antibody (bottom row). Elapsed time is shown in hours. At right: PECAM1-blocking antibodies reduce tube formation by ~50% in PECAM1+PBT2460 cells. Sample means were statistically significant as determined by a Student’st-test (P<0.01). (scale bars, 100 μm, error bars=s.e.m.). Figure 3: PECAM1 + /VEGFR-2 − tumour cells exist in a genetically engineered mouse model of melanoma and they form vascular-like networks in Matrigel. ( a ) Examples of tumours from ΔBraf/Pten −/− mice. ( b ) qPCR analysis of Pecam1 expression in PECAM1 − and PECAM1 + B16F10 clonal populations and two additional unsorted cell lines derived from dispersed tumours from ΔBraf/Pten −/− mice. mEC are a positive control for Pecam1 expression. ( c ) Flow cytometry analysis of unsorted (parental) PBT2460 cells shows ~3% positivity for PECAM1. After six rounds of PECAM1 selection, this fraction increases to ~15% and after eight rounds to ~98%. ( d ) qPCR analysis of the parental PBT2460 population versus the 8X-enriched fraction. Basal Pecam1 expression is ~100-fold higher in the 8X-enriched fraction compared with unsorted PBT2460 cells, whereas neither population expresses VE-cadherin nor Vegfr-2 . ( e ) Using the 8X-enriched fraction, single-cell clones were prepared by limiting dilution assays and then analysed by flow cytometry for PECAM1 expression. ( f ) Clonally derived PECAM1 + PBT2460 cells show an ~5-fold increase in tube formation as compared with PECAM1 − cells. Sample means were statistically significant as determined by a Student’s t -test ( P <0.0001). ( g ) Time-lapse images of tube formation assay using clonally derived PECAM1 + PBT2460 cells incubated with either a nonspecific IgG (top row) or PECAM1-blocking antibody (bottom row). Elapsed time is shown in hours. At right: PECAM1-blocking antibodies reduce tube formation by ~50% in PECAM1 + PBT2460 cells. Sample means were statistically significant as determined by a Student’s t -test ( P <0.01). (scale bars, 100 μm, error bars=s.e.m.). Full size image Using the enriched PECAM1 + fraction from ΔBraf/Pten −/− tumours, we generated single-cell clones by limiting dilution assays. Similar to PECAM1 + tumour cells derived from B16F10, single-cell clones derived from ΔBraf/Pten −/− tumours maintained PECAM1 expression in culture that was detectable on the cell surface by flow cytometry ( Fig. 3e ). Furthermore, clonally derived PECAM1 + tumour cells from ΔBraf/Pten −/− tumours showed a fivefold increase in the formation of vascular-like networks in vitro compared with their PECAM1 − counterparts ( Fig. 3f ). As with B16F10-derived PECAM1 + tumour cells, these tube-like structures were stable over time but could be diminished by ~50% using a PECAM1 neutralizing antibody ( Fig. 3g , Supplementary Movie 1 ). PECAM1 + melanoma cells integrate into vessel lumens in vivo To assess whether PECAM1 + melanoma cells generated vessel-like structures in vivo , we engrafted unlabelled, clonally derived PECAM1 + (clone A5) and PECAM1 − (clone A1) melanoma cells under the skin of C57BL6/J mice. We then stained cryosections with antibodies against PECAM1 and the melanoma marker S100B [36] . Strikingly, in PECAM1 + tumours, we found intratumoural holes and channels lined by PECAM1 + /S100B + tumour cells ( Fig. 4a ). These channels appeared to be formed entirely by PECAM1 + /S100B + tumour cells (top row) or were formed in collaboration with PECAM1 + /S100B + tumour cells and host endothelium (middle row). In contrast, PECAM1 − tumours were characterized by host-derived PECAM1 + vasculature juxtaposed to S100B + tumour cells (bottom row). Next, we used GFP-labelled PECAM1 + and PECAM1 − clonally derived populations from B16F10 to further assess the localization of PECAM1 − and PECAM1 + tumour cells in vivo by immunohistochemistry. Similar to the results above, in PECAM1 + tumours, co-staining using PECAM1 and GFP antibodies revealed large openings, intratumoural channels and vascular-like structures that incorporated GFP + tumour cells within their lumens ( Fig. 4b , first row). In contrast, host-derived PECAM1 + vascular EC were mainly peripheral to GFP + tumour cells in PECAM1 − tumours ( Fig. 4b , second row). We then determined whether PECAM1 + tumour cells were also incorporated into VE-cadherin + vascular lumens. Similar to the staining pattern for PECAM1 above, we found that PECAM1 + tumour cells formed mosaic vascular structures and were incorporated within occasional VE-cadherin + lumens ( Fig. 4b , third row). In contrast, PECAM1 − counterpart tumour cells were localized to the margins of host-derived VE-cadherin + blood vessels ( Fig. 4b , fourth row). Taken together, these results suggest that PECAM1 + melanoma cells have vascular-like properties including the ability to spontaneously organize into tube-like structures in vitro and incorporate into vascular lumens in vivo . 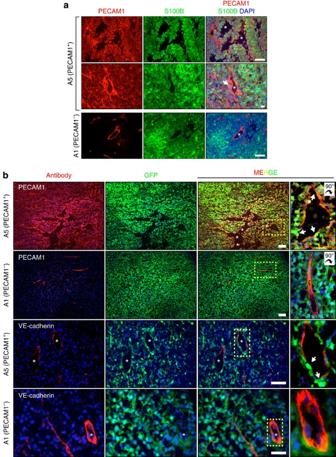Figure 4: PECAM1+melanoma cells integrate within vessel lumensin vivo. (a) Engraftment of unlabelled PECAM1−(clone A1) and PECAM1+(clone A5) tumour cells in C57BL6/J mice. Tumours were implanted subcutaneously and then harvested ~3 weeks later. Frozen sections were stained with PECAM1 and S100b antibodies. Asterisks indicate blood vessels. Arrows show luminally positioned tumour cells. (b) Representative GFP-labelled PECAM1+and PECAM1−tumours are shown. Sections were stained with PECAM1 or VE-Cadherin antibodies where indicated. The boxed regions shown at far right are zoomed regions taken from these images. In the top panels, asterisks indicate tumour cell-lined ‘channels’. The arrows show luminally positioned tumour cells. In the bottom panels, the asterisks and arrows indicate where host-derived VE-cadherin+EC are absent but void space is filled by GFP+/PECAM1+tumour cells. In PECAM1−/GFP+tumours shown for comparison, PECAM1−/GFP+tumour cells surround a host-derived, VE-cadherin+vessel but do not incorporate into the lumen (long scale bars, 100 μm, short, 20 μm). Figure 4: PECAM1 + melanoma cells integrate within vessel lumens in vivo . ( a ) Engraftment of unlabelled PECAM1 − (clone A1) and PECAM1 + (clone A5) tumour cells in C57BL6/J mice. Tumours were implanted subcutaneously and then harvested ~3 weeks later. Frozen sections were stained with PECAM1 and S100b antibodies. Asterisks indicate blood vessels. Arrows show luminally positioned tumour cells. ( b ) Representative GFP-labelled PECAM1 + and PECAM1 − tumours are shown. Sections were stained with PECAM1 or VE-Cadherin antibodies where indicated. The boxed regions shown at far right are zoomed regions taken from these images. In the top panels, asterisks indicate tumour cell-lined ‘channels’. The arrows show luminally positioned tumour cells. In the bottom panels, the asterisks and arrows indicate where host-derived VE-cadherin + EC are absent but void space is filled by GFP + /PECAM1 + tumour cells. In PECAM1 − /GFP + tumours shown for comparison, PECAM1 − /GFP + tumour cells surround a host-derived, VE-cadherin + vessel but do not incorporate into the lumen (long scale bars, 100 μm, short, 20 μm). Full size image PECAM1 + melanoma form perfused vascular structures in mice To determine whether PECAM1 + tumour cells were in direct contact with the host circulation, we examined paraffin-embedded tumour sections stained with GFP antibodies visualized using 3,3′-diaminobenzidine. The results showed numerous channels or ‘lumens’ that were comprised of GFP + tumour cells in direct contact with erythrocytes ( Fig. 5a ). Haematoxylin and eosin (H&E)-stained sections showed large dilated vessels, haemorrhage and blood-filled channels in PECAM1 + tumours versus their PECAM1 − counterparts ( Fig. 5b ). When quantified using the ImageJ software package, the mean haemorrhage area for PECAM1 − tumours was 46.7 ±1.3 AU and 88.3±23.0 AU for PECAM1 + tumours ( Fig. 5b , lower panel). In support of a PECAM1-dependent form of VM in this model, this increase in haemorrhage area was diminished when PECAM1 + tumours were engrafted in PECAM1 KO mice ( Supplementary Fig. 6a–c ). 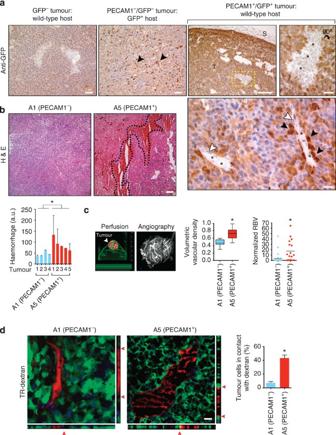Figure 5: PECAM1+melanoma cells form primitive but perfused vascular structures. (a) 3,3′-Diaminobenzidine (DAB) detection of GFP antibodies used to stain tumours. Unlabelled B16F10 tumours implanted in wild-type hosts were used as negative controls. Blood vessels are visible in the centre of field. Unlabelled PECAM1−tumours implanted in a GFP host showed an expected staining pattern of host-derived blood vessels (black arrow heads) and stromal cells. PECAM1+/GFP+tumour cells contained large ‘holes’ and channels, some of which were blood-filled. GFP+tumour cells in right two panels appear to be in direct contact with red blood cells (asterisks). The boxed area in the third panel is magnified on far right. Tumour area is marked with a ‘T’ and the overlying mouse skin (GFP−) is marked with an ‘S.’ Lower panel shows a second PECAM1+clone (clone A2) with PECAM1+/GFP+tumour cells closely aligned with host blood vessels. Some unstained endothelial cell nuclei are also visible and are marked with white arrowheads. (b) H&E-stained sections of PECAM1−and PECAM1+tumours reveals large areas of haemorrhage and vessel dilation. Tumour sections were analysed using ImageJ and are plotted. Sample means were statistically significant as determined by a Student’st-test (P=0.0384,n=5 tumours). (c) Tumour vascularity was measured using three-dimensional acoustic angiography imaging. Means were statistically significant using a Welch two samplet-test (P=0.003,n=9 for PECAM1−tumours andn=8 for PECAM1+tumours). Area-normalized relative blood volume was calculated from two-dimensional destruction-reperfusion imaging. A linear mixed-effects model was used to calculate statistical significance (P=0.0182). (d) TR-Dextran was injected intravenously in mice bearing GFP-labelled PECAM1−or PECAM1+tumours. Harvested tumours were sectioned and imaged on a confocal microscope. Red arrowheads point to GFP+/TR-Dextran+areas. Ten separate fields from tissue sections from each mouse were used to quantify number of tumour cells in contact with the circulation as shown. Means were statistically significant using an unpaired two-tailedt-test, (P<0.0001,n=4; scale bars, 100 μm, short bars in high-magnification panels, 20 μm, error bars=s.e.m.). Figure 5: PECAM1 + melanoma cells form primitive but perfused vascular structures. ( a ) 3,3′-Diaminobenzidine (DAB) detection of GFP antibodies used to stain tumours. Unlabelled B16F10 tumours implanted in wild-type hosts were used as negative controls. Blood vessels are visible in the centre of field. Unlabelled PECAM1 − tumours implanted in a GFP host showed an expected staining pattern of host-derived blood vessels (black arrow heads) and stromal cells. PECAM1 + /GFP + tumour cells contained large ‘holes’ and channels, some of which were blood-filled. GFP + tumour cells in right two panels appear to be in direct contact with red blood cells (asterisks). The boxed area in the third panel is magnified on far right. Tumour area is marked with a ‘T’ and the overlying mouse skin (GFP − ) is marked with an ‘S.’ Lower panel shows a second PECAM1 + clone (clone A2) with PECAM1 + /GFP + tumour cells closely aligned with host blood vessels. Some unstained endothelial cell nuclei are also visible and are marked with white arrowheads. ( b ) H&E-stained sections of PECAM1 − and PECAM1 + tumours reveals large areas of haemorrhage and vessel dilation. Tumour sections were analysed using ImageJ and are plotted. Sample means were statistically significant as determined by a Student’s t -test ( P =0.0384, n =5 tumours). ( c ) Tumour vascularity was measured using three-dimensional acoustic angiography imaging. Means were statistically significant using a Welch two sample t -test ( P =0.003, n =9 for PECAM1 − tumours and n =8 for PECAM1 + tumours). Area-normalized relative blood volume was calculated from two-dimensional destruction-reperfusion imaging. A linear mixed-effects model was used to calculate statistical significance ( P =0.0182). ( d ) TR-Dextran was injected intravenously in mice bearing GFP-labelled PECAM1 − or PECAM1 + tumours. Harvested tumours were sectioned and imaged on a confocal microscope. Red arrowheads point to GFP + /TR-Dextran + areas. Ten separate fields from tissue sections from each mouse were used to quantify number of tumour cells in contact with the circulation as shown. Means were statistically significant using an unpaired two-tailed t -test, ( P <0.0001, n =4; scale bars, 100 μm, short bars in high-magnification panels, 20 μm, error bars=s.e.m.). Full size image Next, we carried out three-dimensional acoustic angiography and dynamic contrast-enhanced perfusion imaging using lipid-encapsulated micro-bubble contrast agents to measure real-time tumour perfusion and vascular structure in PECAM1 − and PECAM1 + tumours ( Fig. 5c , left) [37] . Dual-frequency, three-dimensional acoustic angiography revealed mean volumetric vascular density values of 47.9±2.9 for PECAM1 − tumours, whereas PECAM1 + tumours had mean volumetric vascular density values of 72.3±5.5 ( Fig. 5c , middle). The sample means were statistically significant when analysed using a two-tailed t -test. We observed that the acoustic angiography images showed the presence of greater sub-resolution contrast in PECAM1 + compared with PECAM1 − tumours. This sub-resolution contrast signal likely emanates from pooling blood, which could correspond with the larger haemorrhage areas observed in PECAM1 + tumours. In addition, destruction-reperfusion images acquired longitudinally were used to compute the area-normalized relative blood volume (normalized RBV) analysed using a linear mixed effects model in R. The area-normalized RBV regression intercept was 3.46±2.95U for PECAM1 − tumours and 15.60±4.76U for PECAM1 + tumours, which was statistically significant ( Fig. 5c , right). Overall, these results demonstrate that the normalized RBV of PECAM1 + tumours was an average of 4.5 times higher than that of PECAM1 − tumours. To determine whether PECAM1 + tumour cells were in contact with the circulation, we injected Texas Red-labelled high-molecular-weight Dextran (TR-Dextran) by way of the tail vein in mice bearing PECAM1 − /GFP + or PECAM1 + /GFP + tumours [38] . GFP + tumour cells in direct contact with TR-Dextran were then analysed using confocal microscopy ( Fig. 5d ). After analysing multiple sections from three or four mice per group, we found a sixfold increase in PECAM1 + tumour cells in contact with TR-Dextran when compared with their PECAM1 − counterparts. These results were confirmed in an additional PECAM1 + clone (clone A2; Supplementary Fig. 7a,b , Supplementary Movies 2,3 ). Finally, we carried out transmission electron microscopy of engrafted PECAM1 − and PECAM1 + tumours. The ultrastructure of vessels in these tumours showed melanoma cells (identified by the presence of melanosomes, a unique feature of melanocytes and melanoma cells) in direct contact with the basal lamina of erythrocyte-containing vessels in PECAM1 + tumours, but this contact was rarely seen in PECAM1 − tumours ( Supplementary Fig. 8 ). Thus, these results suggest that PECAM1 + tumour cells organize into primitive vascular channels that may be affiliated with the host circulation and perfused with blood. AP-2α is reduced in PECAM1 + melanoma and represses PECAM1 Next, we asked how PECAM1 expression was transcriptionally regulated in PECAM1 + tumour cells. Notably, we did not find evidence for epigenetic regulation of Pecam1 expression in B16F10 because neither the DNA methyltransferase inhibitor 5-azacytidine (5-Aza) nor the pan-HDAC inhibitor trichostatin A (TSA) could induce Pecam1 mRNA ( Supplementary Fig. 9a ). However, PECAM1 is known to be regulated by the transcription factor GATA2 and additional binding sites in the PECAM1 promoter for SP1, ETS and AP-2α are also reported [39] . We scanned the PECAM1 promoter and used semi-quantitative RT–PCR to measure the expression of these candidate transcription factors in PECAM1 − and PECAM1 + clones. The results showed that unsorted B16F10 melanoma and clonally derived PECAM1 − or PECAM1 + tumour cells either did not express or expressed similar levels of most of these transcription factors, including Ets ( Fig. 6a ). On the other hand, Ap-2α expression was strikingly diminished in PECAM1 + tumour cells and mEC but was expressed in unsorted B16F10 cells and PECAM1 − tumour cells. Ap-2α expression was similar in parental B16F0, the low-metastatic B16 clone B16F1, B16F10 and two independent PECAM1 − clones ( Supplementary Fig. 9b ). Expression of the well-characterized melanoma markers dopachrome tautomerase ( Dct) and micropthalmia-associated transcription factor ( Mitf-m) were also similar in these same cell lines at the mRNA and protein levels ( Supplementary Fig. 9b, c ). Interestingly, PECAM1 + clones consistently produced more pigmented cells in vitro and highly pigmented tumours in vivo despite expressing similar levels of Tyr and Dct compared with PECAM1 − counterparts ( Supplementary Fig. 9d,e ). 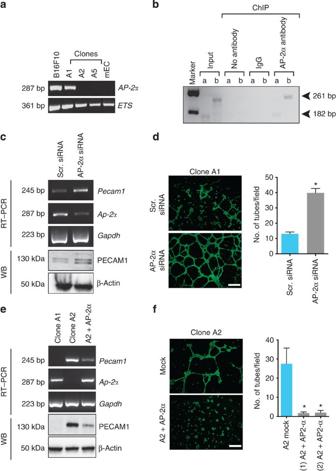Figure 6: AP-2α is diminished in PECAM1+tumour cells and is a transcriptional repressor of PECAM1. (a) Semi-quantitative RT–PCR analysis of Ap-2α and Ets transcription factors in PECAM1−and PECAM1+clones. (b) Chromatin immunoprecipitation using B16F10 tumour cells. Purified genomic DNA was incubated with AP-2α antibodies followed by capture on protein-G agarose. Samples were analysed by semiquantitative RT–PCR using two primer sets predicted to amplify different regions of the mouse Pecam1 promoter (indicated by arrow heads). (c) siRNA knockdown of Ap-2α. Cells were incubated for 48 h with 100 nM of either scrambled control (Scr. siRNA) or Ap-2α siRNA. Cell extracts were then evaluated by RT–PCR and western blotting. (d) Images of tube-forming assay in a PECAM1−clone following Ap-2α siRNA knockdown. Images were taken approximately 16 h after seeding on Matrigel. Quantification of tube-forming ability following Ap-2α siRNA knockdown on right. Results are statistically significant where indicated by an asterisk (P<0.0001 by unpairedt-test,n=12 observations from individual wells). (e) Lentiviral overexpression of Ap-2α in PECAM1+clones. Stable cell lines were established from clonal populations following Ap-2α introduction and selection in Zeocin. Cell extracts were evaluated by RT–PCR and western blotting. (f) Images of tube-forming assay in a PECAM1+clone following Ap-2α lentiviral introduction. Images were taken approximately 16 h after seeding on Matrigel. Quantification of tube-forming ability following Ap-2α lentiviral introduction on right. Results are statistically significant where indicated by an asterisk and were confirmed using two different derived clones (P=0.0202,n=3-4 observations from individual wells; scale bars, 100 μm, error bars=s.e.m.). Figure 6: AP-2α is diminished in PECAM1 + tumour cells and is a transcriptional repressor of PECAM1. ( a ) Semi-quantitative RT–PCR analysis of Ap-2α and Ets transcription factors in PECAM1 − and PECAM1 + clones. ( b ) Chromatin immunoprecipitation using B16F10 tumour cells. Purified genomic DNA was incubated with AP-2α antibodies followed by capture on protein-G agarose. Samples were analysed by semiquantitative RT–PCR using two primer sets predicted to amplify different regions of the mouse Pecam1 promoter (indicated by arrow heads). ( c ) siRNA knockdown of Ap-2α. Cells were incubated for 48 h with 100 nM of either scrambled control (Scr. siRNA) or Ap-2α siRNA. Cell extracts were then evaluated by RT–PCR and western blotting. ( d ) Images of tube-forming assay in a PECAM1 − clone following Ap-2α siRNA knockdown. Images were taken approximately 16 h after seeding on Matrigel. Quantification of tube-forming ability following Ap-2α siRNA knockdown on right. Results are statistically significant where indicated by an asterisk ( P <0.0001 by unpaired t -test, n =12 observations from individual wells). ( e ) Lentiviral overexpression of Ap-2α in PECAM1 + clones. Stable cell lines were established from clonal populations following Ap-2α introduction and selection in Zeocin. Cell extracts were evaluated by RT–PCR and western blotting. ( f ) Images of tube-forming assay in a PECAM1 + clone following Ap-2α lentiviral introduction. Images were taken approximately 16 h after seeding on Matrigel. Quantification of tube-forming ability following Ap-2α lentiviral introduction on right. Results are statistically significant where indicated by an asterisk and were confirmed using two different derived clones ( P =0.0202, n =3-4 observations from individual wells; scale bars, 100 μm, error bars=s.e.m.). Full size image Because AP-2α levels were inversely correlated with PECAM1, we hypothesized that AP-2α might function as a transcriptional repressor of PECAM1. We used chromatin immunoprecipitation (ChIP) to confirm that AP-2α occupied the PECAM1 promoter in B16F10 tumour cells. Immunoprecipitation with an AP-2α antibody followed by PCR using two primer sets unique to the mouse PECAM1 promoter revealed amplified fragments of the predicted sizes ( Fig. 6b ). Furthermore, PECAM1 − tumour cells transfected with Ap-2α short interfering RNA (siRNA) revealed upregulation of Pecam1 mRNA and protein expression, which was accompanied by a fourfold increase in tube formation in Matrigel ( Fig. 6c,d ). On the other hand, stable lentiviral re-expression of Ap-2α into PECAM1 + tumour cells resulted in downregulation of Pecam1 mRNA and protein expression, and a sixfold reduction in tube formation ( Fig. 6e,f , Supplementary Movie 4 ). These results suggest that AP-2α may repress PECAM1 expression and that diminished expression of AP-2α in PECAM1 + B16F10 cells accompanies their ability to form vascular-like structures in vitro . PECAM1 + tumour cells are enriched after anti-VEGF therapy Because PECAM1 + tumour cells do not express VEGFR-2, but engage in VM, we hypothesized they might form VEGF-independent intratumoural channels in mice. First, we subjected mice bearing B16F10-GFP tumours to MCR84, a neutralizing antibody raised against VEGF-A, and then tumours were harvested once they become refractory to further treatment ( Fig. 7a ) [40] , [41] . MCR84-treated mice demonstrated a characteristic delay in tumour growth, followed by tumour regrowth that was resistant to further VEGF inhibition ( Fig. 7b ). We then used flow cytometry to measure the proportion of GFP + /PECAM1 + tumour cells in size-matched tumours. We found that in size-matched, MCR84-resistant tumours, the number of PECAM1 + tumour cells was enriched approximately sixfold, whereas PECAM1 − tumour cells and bona fide EC were marginally reduced ( Fig. 7c,d ). To examine the specific role of PECAM1 + tumour cells in tumour responses to anti-angiogenic therapy, we engrafted GFP-labelled clonally derived populations of either PECAM1 + or PECAM1 − tumour cells into C57BL6/J mice. Mice were then treated with MCR84 as described above. We found that PECAM1 − tumours demonstrated an expected delay in tumour growth and reduction in tumour volume (approximately twofold decrease in tumour volume at day 15) when challenged with MCR84. On the other hand, PECAM1 + tumours showed no appreciable growth inhibition compared with controls ( Fig. 7e ). H&E and GFP-stained tissue sections revealed striking differences in blood vessel morphology and numerous blood-filled ‘channels’ encapsulated by GFP + tumour cells in the PECAM1 + tumours challenged with MCR84 ( Fig. 7f ). Taken together, VEGF blockade induces expansion of a minor subpopulation of PECAM1 + melanoma cells; furthermore, PECAM1 + melanoma cells form tumours that do not respond to VEGF inhibition and they generate aberrant vascular-like structures following challenge with VEGF-blocking antibodies. 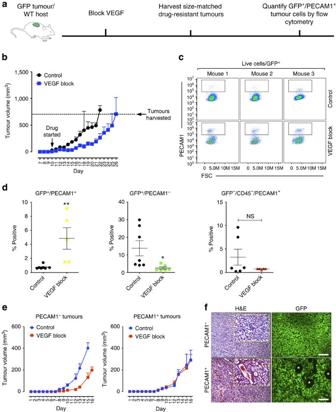Figure 7: PECAM1+tumour cells are enriched in tumours challenged with anti-VEGF therapy. (a) Experimental design. (b) Tumour volumes in control (n=8) and MCR84-treated (n=8) mice measured with calipers each day. MCR84 treatment was initiated where indicated. (c) Flow cytometry analysis of collagenase-dispersed tumours from control and MCR84-treated mice. Three representative dot plots from individual mice are shown. Live cells/GFP+cells were selected and then gated for PECAM1. The top three panels are controls and the bottom three panels are MCR84-treated mice. (d) Quantification of tumour subpopulations from collagenase-dispersed tumours using flow cytometry (n=5–7 mice per group). Results are statistically significant where indicated with an asterisk (left,P=0.0095; centre,P=0.0361; right, NS=not significant) as evaluated by Student’st-test. (e) Tumour growth in mice bearing PECAM1−tumours (clone A1) or PECAM1+tumours (clone A5) challenged with MCR84. Drug treatment was initiated on day 5 and tumour sizes were measured each day with calipers (n=4 or 5 mice per group). (f) H&E- and GFP-stained tissue sections from MCR84-treated PECAM1−and PECAM1+tumours. Zoomed regions (yellow insets) demonstrate dense pockets of PECAM1+tumour cells surrounding a vessel lumen (also identified by asterisks in the accompanying GFP-stained section; scale bars, 100 μm, error bars=s.e.m.). Figure 7: PECAM1 + tumour cells are enriched in tumours challenged with anti-VEGF therapy. ( a ) Experimental design. ( b ) Tumour volumes in control ( n =8) and MCR84-treated ( n =8) mice measured with calipers each day. MCR84 treatment was initiated where indicated. ( c ) Flow cytometry analysis of collagenase-dispersed tumours from control and MCR84-treated mice. Three representative dot plots from individual mice are shown. Live cells/GFP + cells were selected and then gated for PECAM1. The top three panels are controls and the bottom three panels are MCR84-treated mice. ( d ) Quantification of tumour subpopulations from collagenase-dispersed tumours using flow cytometry ( n =5–7 mice per group). Results are statistically significant where indicated with an asterisk (left, P =0.0095; centre, P =0.0361; right, NS=not significant) as evaluated by Student’s t -test. ( e ) Tumour growth in mice bearing PECAM1 − tumours (clone A1) or PECAM1 + tumours (clone A5) challenged with MCR84. Drug treatment was initiated on day 5 and tumour sizes were measured each day with calipers ( n =4 or 5 mice per group). ( f ) H&E- and GFP-stained tissue sections from MCR84-treated PECAM1 − and PECAM1 + tumours. Zoomed regions (yellow insets) demonstrate dense pockets of PECAM1 + tumour cells surrounding a vessel lumen (also identified by asterisks in the accompanying GFP-stained section; scale bars, 100 μm, error bars=s.e.m.). Full size image Human melanoma contains a PECAM1 + subpopulation We examined PECAM1 expression from microarray data generated from >40 human melanoma cell lines and normal human melanocytes [42] . From these data, we identified approximately ten cell lines, which fell above a threshold (~1.5 adjusted mean fluorescence values from microarray data) established using normal human melanocytes, which do not express PECAM1 ( Fig. 8a ). A list of normal melanocytes and melanoma cells along with the raw fluorescence values from the microarray are shown in Supplementary Table 2 . We began by culturing some of the highest PECAM1-expressing cell lines and measuring PECAM1 mRNA levels by quantitative RT–PCR. The results showed that, as predicted from the microarray analysis, PECAM1 mRNA was detected in the WM2664, MEL505, RPMI7951, WM1158 and SBCl2 cell lines, albeit at very low levels compared with human EC ( Fig. 8b ). No PECAM1 transcripts were detected in normal melanocytes, RPMI8332 or SKMEL119, which all fell below the established threshold on the microarray. On the other hand, VE-CADHERIN mRNA, which is expressed in some uveal forms of melanoma that engage in VM, was not detected in most cell lines but was found at very low levels in WM1158 cells [43] . Using flow cytometry, we could detect a minor shift in PECAM1 fluorescence in RPMI7951 (3.3%) and WM1158 cells (1.6%) but a much larger shift in SBCl2 cells (50%). No PECAM1 surface expression was detected in normal melanocytes (NHM7) or in RPMI8332, as expected ( Fig. 8c ). Similar to the PECAM1 + fractions derived from murine B16F10 and ΔBraf/Pten −/− cells, SBCl2 melanoma cells formed robust and stable vessel-like networks in vitro, which were inhibited by PECAM1 neutralizing antibodies ( Fig. 8d , Supplementary Movie 5 ). 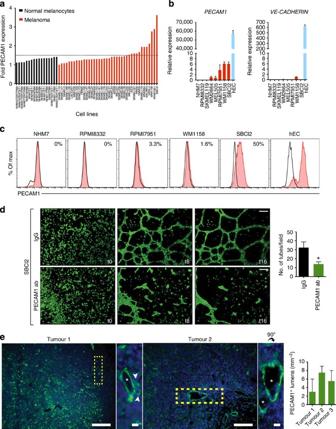Figure 8: Human melanoma contains a PECAM1+subpopulation that displays vascular-like characteristics. (a) Microarray analysis of normal human melanocytes (black bars) and human melanoma (red bars). Each cell line and the raw fluorescence intensity value from the microarray are listed inSupplementary Table 2. The dotted horizontal line on the graph is the threshold below which noPECAM1transcripts are detected. (b) Quantitative real-time PCR analysis of PECAM1 and VE-CADHERIN expression in normal melanocytes and seven of the highestPECAM1-expressing cell lines predicted from the microarray. Except for WM1158, no VE-CADHERIN transcripts were detected. Human endothelial cells (hECs) were used as a positive control. (c) Flow cytometry of selected cell lines stained with human-specific PECAM1 antibodies. (d) Time-lapse images of tube formation assay using the PECAM1+human melanoma cell line SBCl2 incubated with either a nonspecific IgG (top row) or a PECAM1-blocking antibody (bottom row). Far right: PECAM1-blocking antibodies reduce tube formation by ~60% in PECAM1+SBCl2 cells. Sample means were statistically significant as determined by a Student’st-test (P=0.02,n=8 wells per condition). (e) PECAM1+lumens formed by SBCl2 tumours. The asterisks mark lumens and white arrow head shows PECAM1+tumour cells positioned at the abluminal surface. Two sections from each tumour were scanned for PECAM1+lumens and the mean values were plotted on right (scale bars, 100 μm, short bars in high-magnification panels, 20 μm, error bars=s.e.m.). Figure 8: Human melanoma contains a PECAM1 + subpopulation that displays vascular-like characteristics. ( a ) Microarray analysis of normal human melanocytes (black bars) and human melanoma (red bars). Each cell line and the raw fluorescence intensity value from the microarray are listed in Supplementary Table 2 . The dotted horizontal line on the graph is the threshold below which no PECAM1 transcripts are detected. ( b ) Quantitative real-time PCR analysis of PECAM1 and VE-CADHERIN expression in normal melanocytes and seven of the highest PECAM1 -expressing cell lines predicted from the microarray. Except for WM1158, no VE-CADHERIN transcripts were detected. Human endothelial cells (hECs) were used as a positive control. ( c ) Flow cytometry of selected cell lines stained with human-specific PECAM1 antibodies. ( d ) Time-lapse images of tube formation assay using the PECAM1 + human melanoma cell line SBCl2 incubated with either a nonspecific IgG (top row) or a PECAM1-blocking antibody (bottom row). Far right: PECAM1-blocking antibodies reduce tube formation by ~60% in PECAM1 + SBCl2 cells. Sample means were statistically significant as determined by a Student’s t -test ( P =0.02, n =8 wells per condition). ( e ) PECAM1 + lumens formed by SBCl2 tumours. The asterisks mark lumens and white arrow head shows PECAM1 + tumour cells positioned at the abluminal surface. Two sections from each tumour were scanned for PECAM1 + lumens and the mean values were plotted on right (scale bars, 100 μm, short bars in high-magnification panels, 20 μm, error bars=s.e.m.). Full size image Because SBCl2 expressed detectable PECAM1 levels by flow cytometry, we engrafted this cell line subcutaneously in NOD-SCID-γ (NSG) mice. We then stained primary, paraffin-embedded SBCl2 tumours with PECAM1 antibodies that were verified to be human specific using western blotting and immunohistochemistry ( Supplementary Fig. 10a,b ). Although the majority of PECAM1 + tumour cells detected with human antibodies appeared randomly scattered throughout the tumour, occasional PECAM1 + ‘lumens’ were also visible ( Fig. 8e ). Overall, PECAM1 + tumour cells were found at the luminal and abluminal surface of vascular structures (white arrowheads), were detected in all SBCl2 tumours examined, and were present at an average density of ~5 vessel-like structures per mm 2 when normalized to tumour size for each tissue section ( Fig. 8e , far right). Thus, similar to mouse melanoma, a subpopulation of some human melanoma cells express PECAM1 and engage in the formation of vascular-like structures in vitro and in vivo . We have identified a subpopulation of PECAM1 + melanoma cells that was ‘hidden’ within heterogeneous and predominantly PECAM1 − melanoma tumours. Generally, PECAM1 + melanoma cells were more motile and coalescent in Matrigel, which could be reversed by introduction of the AP-2α transcription factor. However, PECAM1 expression was only partially repressed upon AP-2α introduction, indicating additional factors regulate PECAM1 expression in melanoma cells. Furthermore, the nature of the AP-2α defect in PECAM1 + tumour cells is not yet clear and its diminished expression in these cells could be due to mutations, epigenetic silencing or other unknown mechanisms. AP-2α is a putative tumour suppressor shown to act as a transcriptional repressor of melanoma cell adhesion molecule (MCAM) and activator of KIT [44] , [45] . AP-2α also controls melanoma cell motility and its expression is diminished in aggressive forms of melanoma and breast cancer [46] , [47] . Consistent with a role for AP-2α in cellular movement, we found that introduction of AP-2α into PECAM1 + tumour cells completely blocked in vitro tube formation, a process involving cellular migration and stable intercellular connections. PECAM1 + tumour cells were present within the B16F10 population in low abundance, and we were unable to detect PECAM1 expression in the low-metastatic B16 clone B16F1. However, it is possible that an infrequent population of VM-competent tumour cells could also be enriched from these cell lines in nascent tumours or at sites of metastasis. For example, a minor population of PECAM1 + tumour cells could assist during initial tumour neovascularization (when tumours are relatively small and have yet to recruit an efficient blood supply) by forming transient vascular channels that conduct blood or fluid. Remarkably, this concept was first suggested over 40 years ago in studies using melanoma transplants in the hamster cheek pouch [48] . It is also possible that not all ‘channels’ formed by PECAM1-lined structures contain flowing blood and may thus resemble ‘blood lakes’ described previously [49] . Whether or not these ‘blood lakes’ are inert reservoirs or play an active, pathophysiological role in tumour progression remains unclear. VM-competent tumour cells could also be generated because of selection pressure (differentiation from PECAM1 − counterparts) or mobilized in tumours challenged with angiogenesis inhibitors. Indeed, we found an approximately sixfold enrichment of PECAM1 + tumour cells in B16F10 tumours challenged with the VEGF-blocking antibody, MCR84. PECAM1 + /VEGFR-2 − tumour cells could therefore supplant vascular EC lost following treatment with anti-angiogenic therapy and form PECAM1-dependent ‘bridges’ between neighbouring tumour cells and EC ( Fig. 9a,b ). 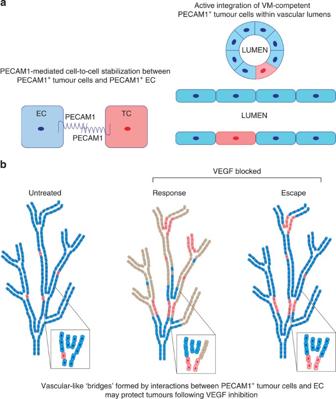Figure 9: A model for a PECAM1-dependent form of vasculogenic mimicry. (a) PECAM1 plays a well-characterized role in stabilizing junctions between EC and leukocytes and between two EC. Tumour cell expression of PECAM1 may also stabilize interactions between tumour cells (TC) and EC or between two PECAM1+TC to form stable junctions. (b) In tumours where PECAM1+tumour cells are present, VEGF-independent ‘bridges’ would not be affected by anti-VEGF therapies and could supplant host endothelium following VEGF inhibition. ‘Channels’ formed exclusively by PECAM1+TC could also be insensitive to VEGF blockade. Figure 9: A model for a PECAM1-dependent form of vasculogenic mimicry. ( a ) PECAM1 plays a well-characterized role in stabilizing junctions between EC and leukocytes and between two EC. Tumour cell expression of PECAM1 may also stabilize interactions between tumour cells (TC) and EC or between two PECAM1 + TC to form stable junctions. ( b ) In tumours where PECAM1 + tumour cells are present, VEGF-independent ‘bridges’ would not be affected by anti-VEGF therapies and could supplant host endothelium following VEGF inhibition. ‘Channels’ formed exclusively by PECAM1 + TC could also be insensitive to VEGF blockade. Full size image We found that PECAM1-blocking antibodies could reduce the tube-forming ability of PECAM1 + tumour cells as they do in cultured EC [31] . Notably, PECAM1 introduction into mesothelioma cells (which do not express PECAM1) also induces robust tube formation in Matrigel [32] . PECAM1 is required for tube formation in bona fide EC, whereas VE-cadherin mediates both cell–cell adhesion and vacuole fusion [50] . Thus, PECAM1 expression in melanoma may mediate cell elongation, migration and invasion while stabilizing the junctional, homophilic complexes between neighbouring cells necessary to create a patent lumen [51] . Taken together, our model is rather different from a passive process of tumour cell-to-EC mosaicism observed in other tumour types [52] , [53] . Instead, co-option of PECAM1 by tumour cells may actively stabilize cell–cell interactions between PECAM1 + tumour cells and between PECAM1 + tumour cells and EC. PECAM1 is typically concentrated at cell–cell borders by a process known as ‘diffusion trapping’, which leads to cell aggregation where two PECAM1 + cells meet [54] . Indeed, homophilic PECAM1-PECAM1 binding was suggested, many years ago, to mediate in vitro tumour cell adhesion to EC in co-culture studies [55] . Given the role of PECAM1 in mediating diapedesis (transendothelial migration) by inflammatory cells, it may be interesting to revisit recent studies demonstrating distinct mechanisms of metastasis using the B16F10 model to determine whether subpopulations of PECAM1 + tumour cells are involved [56] . We found PECAM1 tyrosine phosphorylation in melanoma cells, suggesting PECAM1-mediated signal transduction could function analogously in EC and in PECAM1 + melanoma cells. In support of this possibility, clonal populations of PECAM1 + melanoma displayed a slight growth delay compared with PECAM1 − counterparts suggesting that PECAM1-PECAM1 interactions between tumour cells could stimulate contact inhibition, as it does in EC, and a slower rate of growth despite their ability to form vascular-like channels in vivo . It is therefore possible that acquisition of vascular-like characteristics by tumour cells could come at the expense of reduced tumorigenicity overall. Taken together, the PECAM1 + population of melanoma cells we have uncovered could play multiple roles in diverse processes related to melanoma development, dormancy, migration/invasion and angiogenesis. Mice For studies using the B16F10 melanoma cell lines, female C57BL6/J mice were used (Jackson Laboratories). Mice were injected with tumour cells at 7–8 weeks of age. For engraftment of human melanoma cells, we used female NSG mice (7–8 weeks of age) provided by the mouse phase I unit at University of North Carolina (UNC). C57BL/6-Tg (CAG-EGFP) 1Osb/J mice were purchased from Jackson Laboratories. Pecam1 knockout mice were kindly provided by Dr E. Tzima (UNC, Chapel Hill), and tumour cells were engrafted in female mice at 7–8 weeks of age. All mouse experiments were carried out in accordance with protocols approved by the Institutional Animal Care and Use Committee at the UNC at Chapel Hill. Cell lines and media B16F0, B16F1, B16F10 (American Type Culture Collection (ATCC)), ΔBraf/Pten −/− (derived from B6.Cg-Braf tm1Mmcm Pten tm1Hwu Tg (Tyr-cre/ERT2) 13Bos/BosJ mice (UNC-Chapel Hill Mouse Phase 1 Unit)) cell lines PBT2460 and PBT2130 (Drs W. Kim and J. Bear, UNC-Chapel Hill), and human melanoma cell lines WM1158, SBCl2, Sk-Mel-119, Sk-Mel-173 and WM2664 (Dr J. Shields, UNC-Chapel Hill) were maintained in DMEM with 4.5 g ml −1 D -glucose and 10% FBS. Human melanoma cell lines RPMI7951, RPMI8322 and Mel505 (Dr J Shields, UNC-Chapel Hill) were maintained in RPMI with 10% FBS. The normal human melanocyte line NHM7 (Dr J Shields, UNC-Chapel Hill) was maintained in Media 254 (Gibco) supplemented with HGMS (Gibco). EC (isolated by us previously [8] ) were maintained in Endothelial Cell Media (EC-Media), composed of DMEM with 1 g l −1 glucose, 5 μg l −1 basic FGF (bFGF), 10 μg l −1 VEGF, 100 mg l −1 heparin, antibiotics, and 10% NuSerum IV (BD). Antibodies For a complete list of antibodies and dilutions used, please refer to Supplementary Table 3 . Western blotting Whole-cell lysates were prepared in radioimmunoprecipitation assay buffer (Boston BioProducts), separated by SDS–PAGE at 100 V using a Bio-Rad 4–20% TGX gel (Bio-Rad), blocked with 5% Milk-TBS-T for standard western blotting, 5% BSA for phospo-VEGFR2 blotting and probed with antibodies overnight at 4 °C. Peroxidase-conjugated secondary antibodies were incubated at room temperature for 1 h, and bands were exposed with Western Lightning (PerkinElmer). Blots were imaged on a Fluorchem M (ProteinSimple). All antibodies and dilutions are presented in Supplementary Table 3 . Uncropped western blots are presented in Supplementary Fig. 11 . Chromatin immunoprecipitation ChIP experiments were performed using the ChIPit Express Kit (Active Motif) according to the manufacturer’s instructions. Two micrograms of anti-AP-2α antibodies were used for immunoprecipitation and bound DNA was analysed using two primer sets designed against the mouse PECAM1 promoter (for sequences see Supplementary Table 1 ). siRNA knockdown Cells were plated at 2.0 × 10 5 cells per well in six-well plates. siRNA SmartPools (Dharmacon) targeting Ap-2α (M-062788-01-0005), Pecam1 (TRC RMM4534-EG18613) or non-targeting controls (D-001206-13-05) were added to plates the next day according to the manufacturer’s instructions at a concentration of 100 nM. Cells were allowed to grow for 48 h before harvesting. Isolation of PECAM1 + tumour cells Tumours were harvested and prepared for cell isolation as previously described by us [8] , [57] . In brief, tumours were minced in cold DMEM with 1 g l −1 glucose. Tumours were further digested using a mechanical tissue homogenizer (Miltenyi). Samples were incubated at 37 °C with 5 ml Collagenase T2 (2 mg ml −1 , Worthington), 1 ml neutral buffered protease (2.5 U ml −1 , Worthington) and 75 μl deoxyribonuclease (1 mg ml −1 , Worthington) for 75 min. Red blood cells (RBCs) were lysed with 1 × Pharmlyse B (BD PharMingen). Cells were suspended in FACS Buffer (degassed phosphate-buffered saline containing 2 mM EDTA and 0.5% BSA), Fc receptors were blocked with Fc Block (Miltenyi) and 10 μg PE-conjugated anti-PECAM1 antibodies were added for 20 min. Cells were washed and resuspended with anti-PE magnetic beads (Miltenyi) for 15 min. Cells were then washed and passed over a magnetic column, washed and then eluted. Eluted cells were washed and plated in EC-Media. Cells were grown for several weeks, and the isolation was repeated until cultures reached ~99% PECAM1 positivity, at which point single-cell clones were made by limiting dilutions. Tumour dissociation and flow cytometry Single-cell suspensions were prepared either from whole tumours as described above or from detached cell cultures as previously described by us [57] . Briefly, cells were washed with PBS and detached using accutase (Sigma) and then labelled with fluorophore-tagged antibodies. Cells were then washed and fixed in FACS buffer containing 1% paraformaldehyde. Cells were analysed by flow cytometry using an Accuri C6 flow cytometer running BD Accuri CFlow Plus Analysis software. Samples were then analysed using the FloJo software package (version 10). Immunohistochemistry Tumours were harvested and fixed in 4% paraformaldehyde overnight at 4 °C. Samples were then cryoprotected in 30% sucrose overnight. Samples were frozen in OCT and cut into 7 μm sections. Slides were fixed in methanol for 20 min, and washed in PBS. Sections were blocked in 5% BSA with species-specific serum (5%) for 1 h, and antibodies were added in blocking buffer. All antibodies and dilutions are described in Supplementary Table 3 . Slides were incubated overnight at 4 °C. Slides were washed and secondary antibodies were added for 1 h at room temperature. Slides were counterstained with Vectashield Hard-set Mounting Medium with DAPI (Vector Labs). Sections were analysed on a Leica DM-IRB inverted microscope or a Zeiss 710 laser scanning confocal microscope. Images were globally adjusted using ImageJ analysis software ( http://rsb.info.nih.gov/ij ) to enhance contrast and sharpness. Acoustic angiography and perfusion imaging Two methods of contrast-enhanced ultrasonography were employed to quantify perfusion in PECAM1 + and PECAM1 − tumours in vivo . In addition, non-contrast ultrasound provided reference anatomical information and tumour volume. The lipid encapsulated microbubble contrast agents were prepared with a (9:1) molar mixture of 1,2-distearoyl-sn-glycero-3-phosphocholine (Avanti Polar Lipids), and 1,2-distearoyl- sn -glycero-3-phosphoethanolamine- N -methoxy(polyethylene glycol)-2000 (Creative PEGWorks) in phosphate-buffered saline containing 15% (v/v) propylene glycol and 5% (v/v) glycerol. Air in the headspace (1.5 ml in a 3 ml vial) was exchanged with decafluorobutane (SynQuest Labs), and microbubbles were created by agitation with a Vialmix mixer (Bristol-Myers Squibb Medical Imaging) [58] . Activated microbubbles were diluted and injected intravenously through a tail-vein catheter at a rate of 2.8 × 10 7 bubbles per min. Destruction-reperfusion imaging was performed using a Vevo 2100 ultrasound system (VisualSonics) and dynamic contrast-enhanced perfusion imaging sequences were used to compute RBVs (VevoCQ-Advanced Contrast Quantification Software Analysis Tool for the Vevo 2100, VisualSonics, © Bracco Suisse S.A. 2010) [59] . Data were normalized by tumour cross-sectional areas as defined by regions of interests (ROIs) drawn manually. Acoustic angiography utilizes a prototype dual-frequency transducer, with a low frequency element to transmit at 4 MHz, exciting microbubbles to produce broadband, superharmonic echoes (at a mechanical index of 0.6). The confocal high-frequency element (30 MHz) is used to receive the microbubble response, thus avoiding tissue signal and producing high-contrast, high-resolution images of the tumour microvasculature without tissue background, in three dimensions [37] . Acoustic angiography is acquired near simultaneously with b-mode soft tissue imaging, which provides anatomical reference. These images were used to compute the volumetric vascular density of the tumours using the following procedure in MATLAB (MathWorks Inc.). First, ROIs were drawn manually to define tumour boundaries based on the b-mode images. Then, the ROIs were applied to mask the tumour volume in the acoustic angiography images. Finally, the vascular volume was computed by applying an intensity threshold cutoff, to segment the image into vascular and nonvascular regions. The volumetric vascular density is the ratio of the number of voxels classified as vascular volume over the total number of voxels in the tumour ROI. Statistical analysis was carried out using R ( http://www.R-project.org ). Transmission electron microscopy PECAM1 + or PECAM1 − tumours were grown as described above. Tissues were harvested, fixed in 2.5% glutaraldehyde/2% paraformaldehyde (PFA) in 0.15 M sodium phosphate buffer. Samples were post-fixed for 1 h in 1% osmium tetroxide in 0.15 M sodium phosphate buffer, dehydrated with a graded series of ethanol washes, treated with propylene oxide and embedded in PolyBed 812 epoxy resin (Polysciences). Ultrathin sections (70–80 nm) were cut and mounted on copper grids and stained with 4% aqueous uranyl acetate and Reynolds’ lead citrate. Sections were mounted to copper grids, OsO 4 was used to stain the tissues and sections were imaged on a Zeiss Leo EM910 TEM. Lentiviral constructs and transduction All recombinant DNA work was carried out under approval of the Environmental Health Safety Division of UNC-Chapel Hill. Lentiviral expression plasmids were created by E. Campeau and obtained from Addgene: pLenti CMV-GFP-DEST (736-1, Addgene plasmid 19732), pLenti CMV/TO GFP-Zeo DEST (719-1, Addgene 17431). Packaging plasmids psPax2 and pMD2.6 were created by Didier Trono (Addgene plasmids 12259 and 12260). Mouse ORF-eome constructs were acquired from the ATCC I.M.A.G.E Consortium, then cloned into pDONR 221 (Invitrogen) Gateway donor vectors using Clonase BP (Invitrogen). Cloned pDONR 221 vectors were sub-cloned into lentiviral expression vectors by Clonase LR reaction (Invitrogen). Lentiviral backbones were transfected with 1.5 μg packaging plasmids psPAX2 and pMDG2 with 15 μl Lipofectamine 2000 in six-well plates into HEK293T cells. Viral particles were harvested at 24 and 48 h post transfection. Viral particles were used to infect target cells with 10 μg ml −1 Polybrene in antibiotic-free media. Tumour studies in mice B16F10 melanoma cells were grown in appropriate culture medium, detached and resuspended in HBSS (Gibco). 1.0 × 10 6 tumour cells were injected subcutaneously in the right shoulder of C57BL6/J mice. Tumours were allowed to grow to 1 cm 3 and were measured daily with calipers. For MCR84 studies, mice were treated intraperitoneally every other day with 25 mg kg −1 day −1 MCR84 or isotype control antibodies as previously described [41] , [60] . Tumour sizes were measured with calipers each day. At the end of the experiment, mice were euthanized and tumours were harvested and weighed. Microarray analysis RNA was harvested from cell lines and run on a Mouse Gene ST1.0 Chip (Affymetrix). Heat maps were generated using the Gene-E software package, version 2.1.134. ( http://www.broadinstitute.org/cancer/software/GENE-E/ ). Polymerase chain reaction Primers were designed using Invitrogen Primer Perfect Design Software (Invitrogen). End-point PCR was completed using a standard PCR kit (NEB). RT-qPCR was completed with Maxima SYBR Green (ThermoFisher) on an Applied Biosystems Step One Plus analyzer (Applied Biosystems). All qPCR experiments were run in triplicate and data are presented as the average with the standard error of the mean (s.e.m.). Primer sequences used are presented in Supplementary Table 1 . Tumour haemorrhage quantification H&E-stained sections were imaged using polarized light microscopy, which caused RBCs to fluoresce. Images were subsequently converted to a binary image using ImageJ software. The images were then thresholded to only show RBCs and the ‘count particles’ tool was used to analyse RBC content. The first 500 observations were binned and plotted. In vitro tube-forming assays Briefly, 50 μl Matrigel (BD) was plated in 96-well culture dishes and allowed to polymerize at 37 °C for 30 min. Next, 2.5 × 10 4 cells per well were plated on the Matrigel layer and grown for 16 h. Randomized fields were captured using a DM-IRB inverted microscope and tubes were quantified from each image. Data are presented as the average number of tubes per field ±s.e.m. from multiple fields. For live imaging experiments, Matrigel was plated in 24-well plates, and 5 × 10 4 cells per well were seeded on top of the layer. Tube formation was imaged on a Leica IX70 microscope outfitted with an environmental chamber. Data were compiled using ImageJ Analysis Software. Brightfield images were converted to eight-bit black and white and the ‘find edges’ command was used to identify cells. Images were enhanced using sharpen tools and pseudocoloured for video analysis. Dextran perfusion Dextran perfusion was carried out according to the previously published methods [38] . GFP-labelled tumour cells were injected subcutaneously as described. Once tumours reached 1 cm 3 , mice were injected with 100 μl, 70 kD Texas Red Dextran (Life Technologies) via the tail vein and killed 3 min post injection. Tumours were prepared for immunohistochemistry as described and imaged with a Zeiss LSM700 scanning laser confocal microscope. Tumour-cell affiliated dextran was quantified by identifying GFP + cells abutting on dextran-lined channels in tumours and are presented as average tumour cells integrated within lumens per field. XTT assay XTT Assay Kit (ATCC) was used to measure growth of cells. 5,000 cells were plated in triplicate in a 96-well plate. XTT reagent was prepared per manufacturer’s recommendations, added to wells and absorbance at 475 nm was measured after 4 h. 5-Aza and TSA treatment 5-Aza (stock: 819 mM) or TSA (stock: 6.6 mM) were diluted as indicated and added to media. Cells were harvested 7 days later and RNA was purified for semi-quantitative RT–PCR analysis. Karyotypes Cells were treated with 0.1 μg ml −1 colcemid (Irvine Scientific) for 3 h to accumulate cells in metaphase. Cells were then treated with hypotonic 0.075 M KCl for 25 min at 37 °C and fixed in 3:1 methanol/acetic acid. Air-dried slides were stained for G-band analysis and at least 20 metaphase cells were counted for each cell line by the Brigham and Women’s Hospital CytoGenomics Core Laboratory, Boston, MA, USA. Statistical analysis Statistical power for mouse experiments was calculated using Biomath (biomath.info/power). All samples sizes were equal to or greater than recommended minimum group size. All measurements in mouse studies were done with the assistance of at least one blinded researcher for recording and confirmation. Statistical analysis was carried out using the Graphpad Prism 5.0f statistical analysis package unless otherwise noted. Figure legends list specific n and P values. Data are presented as mean±standard error of the mean (s.e.m. ). Accession codes : Microarray data are available at the Gene Expression Omnibus, accession number: GSE59564 . How to cite this article: Dunleavey, J. M. et al. Vascular channels formed by subpopulations of PECAM1 + melanoma cells. Nat. Commun. 5:5200 doi: 10.1038/ncomms6200 (2014).